Reelin delays amyloid-beta fibril formation and rescues cognitive deficits in a model of Alzheimer’s disease Reelin is an extracellular matrix protein that is crucial for neural development and adult brain plasticity. While the Reelin signalling cascade has been reported to be associated with Alzheimer’s disease (AD), the role of Reelin in this pathology is not understood. Here we use an in vitro approach to show that Reelin interacts with amyloid-β (Aβ 42 ) soluble species, delays Aβ 42 fibril formation and is recruited into amyloid fibrils. Furthermore, Reelin protects against both the neuronal death and dendritic spine loss induced by Aβ 42 oligomers. In mice carrying the APP Swe/Ind mutation (J20 mice), Reelin overexpression delays amyloid plaque formation and rescues the recognition memory deficits. Our results indicate that by interacting with Aβ 42 soluble species, delaying Aβ plaque formation, protecting against neuronal death and dendritic spine loss and preventing AD cognitive deficits, the Reelin pathway deserves consideration as a therapeutic target for the treatment of AD pathogenesis. Characterized by progressive cognitive deficits, synaptic loss and severe neurodegeneration, Alzheimer’s disease (AD) is the most common form of dementia in the elderly. At the histopathological level two main hallmarks have been described, namely neurofibrillary tangles (intracellular bundles of hyperphosphorylated Tau) and senile plaques (extracellular deposits of amyloid-β (Aβ) peptide) [1] , [2] . Aβ peptides are generated by the endoproteolysis of the transmembrane protein amyloid precursor protein (APP), a process performed by the sequential action of β- and γ-secretase complexes. A diversity of Aβ peptides, varying in length depending on the specific cleavage site, are released extracellularly, the 42-residue-long form (Aβ 42 ) being among the most pathogenic [3] . Aβ peptide aggregates into toxic oligomeric species, which are considered to be responsible for the synaptic failure in AD [4] , [5] , [6] , [7] , [8] . The aggregation process ends with the formation of amyloid fibrils, the major constituents of the plaques. AD combines its own specific underlying pathogenic mechanisms with a common gradual failure of neuroprotective mechanisms [9] . Therapeutic strategies aiming at ameliorating AD have not been effective so far [10] . Therefore strengthening the pathways that homeostatically regulate global neuronal function in the adult brain may be a useful therapeutic strategy for AD. Reelin is an extracellular matrix protein that is crucial for neural development and it is also expressed in the adult cerebral cortex [11] , [12] . Through the regulation of development-reminiscent mechanisms, Reelin increases hippocampal neurogenesis and promotes synaptic plasticity by enhancing structural and functional properties at the synapse [13] . In relation to AD pathology, Reelin is present in amyloid plaques [14] , controls APP processing [15] , reduces Tau phosphorylation by inhibiting GSK3β [16] and counteracts Aβ-induced synaptic dysfunction [17] . In addition, AD brain samples show altered levels of Reelin [18] , [19] , [20] , [21] , [22] , and the RELN gene bears polymorphic variants associated with normal cognitive function in AD pathology [23] , [24] . Finally, the reduction of Reelin in an AD mouse model accelerates the onset of plaque formation and Tau pathology [25] . Here, we address the role of Reelin in Aβ pathology, focusing both on its effect on Aβ aggregation and on Aβ species-mediated toxicity. Moreover, to analyse the effect of Reelin levels in an in vivo model of AD pathology, we cross-breed conditional transgenic mice overexpressing Reelin (TgRln) [13] with mice overexpressing hAPP Swe/Ind (J20) [26] . We find that Reelin delays fibril formation—by interacting with Aβ 42 soluble species—until it is sequestered into amyloid fibrils. Importantly, we show that Reelin overcomes the toxicity of Aβ oligomers, rescues dendritic spine density in J20 mice and enhances cognitive performance in both aged wild-type and J20 mice. Reelin delays Aβ fibrillization and extends oligomer lifetime To monitor the effects of Reelin on Aβ 42 aggregation, we developed a chromatographic protocol to efficiently obtain purified recombinant Reelin. Supernatants from 293T cells stably transfected with Reelin or GFP (Mock control) were subjected to anion exchange chromatography ( Fig. 1a ). Collected peaks were subsequently subjected to size exclusion chromatography ( Fig. 1b ), obtaining Reelin and Mock purified samples ( Fig. 1c ). Biological activity of purified Reelin was assessed by analysing the phosphorylation levels of the Reelin transducer Dab1 after incubation of forebrain neuronal cultures with Reelin preparations ( Fig. 2a,b ) [27] , [28] . 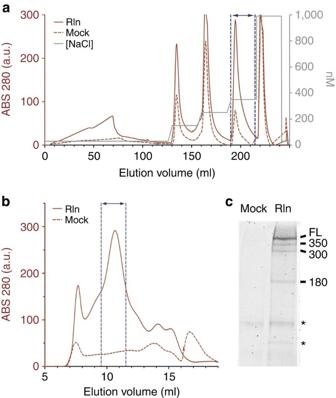Figure 1: Reelin purification. (a) Anion exchange (ANX) chromatogram of supernatants from 293T cells stably transfected with Reelin (Rln) or GFP (Mock). Reelin and Mock elution profiles are represented by a red continuous and a red dashed curve respectively. The grey line represents the mobile phase elution gradient. Reelin peak and the correspondent Mock fractions are delimited by violet dashed lines. (b) Size exclusion chromatogram of ANX-Reelin/Mock-collected peaks. Reelin and Mock elution profiles are represented by a red continuous and a red dashed curve, respectively. Reelin peak and the correspondent Mock fractions, delimited by violet dashed lines, are used as purified samples forin vitrostudies. (c) Purified Reelin and Mock control were subjected to SDS-PAGE, followed by Sypro Ruby staining. Full-length (FL) Reelin and its 350-, 300- and 180-kDa fragments are indicated. Asterisks indicate non-specific proteins coming from the cell supernatant. Figure 1: Reelin purification. ( a ) Anion exchange (ANX) chromatogram of supernatants from 293T cells stably transfected with Reelin (Rln) or GFP (Mock). Reelin and Mock elution profiles are represented by a red continuous and a red dashed curve respectively. The grey line represents the mobile phase elution gradient. Reelin peak and the correspondent Mock fractions are delimited by violet dashed lines. ( b ) Size exclusion chromatogram of ANX-Reelin/Mock-collected peaks. Reelin and Mock elution profiles are represented by a red continuous and a red dashed curve, respectively. Reelin peak and the correspondent Mock fractions, delimited by violet dashed lines, are used as purified samples for in vitro studies. ( c ) Purified Reelin and Mock control were subjected to SDS-PAGE, followed by Sypro Ruby staining. Full-length (FL) Reelin and its 350-, 300- and 180-kDa fragments are indicated. Asterisks indicate non-specific proteins coming from the cell supernatant. 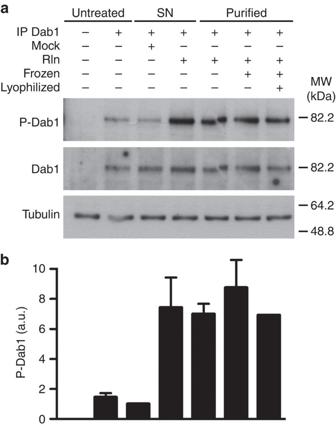Figure 2: Analysis of purified Reelin biological activity. Reelin biological activity is assessed as the ability to induce phosphorylation of Dab1 after treatment of mouse neuronal primary cultures. (a) Phosphorylation of Dab1 is detected by immunoprecipitation (IP) of total Dab1 followed by western blot (WB) anti-phosphotyrosines. Negative control of IP and basal levels of Dab1 phosphorylation are shown respectively in lanes 1 and 2. Mock sample does not induce changes in the basal levels of Dab1 phosphorylation (Lane 3). Reelin supernatants induce a high increase in the phosphorylation of Dab1 (Lane 4). Purified Reelin is also functional (Lane 5) and maintains its activity after nitrogen freezing and lyophilization (Lanes 6 and 7). (b) Densitometric analysis of phosphorylated Dab1 WB images shows a 6–8-fold increase upon Reelin treatment in one to three independent experiments (n=3 for lanes 2–4;n=2 for lanes 1,5 and 6 andn=1 for lane 7). Full-size blots can be found inSupplementary Fig. 1. Data are represented as mean±s.e.m. Full size image Figure 2: Analysis of purified Reelin biological activity. Reelin biological activity is assessed as the ability to induce phosphorylation of Dab1 after treatment of mouse neuronal primary cultures. ( a ) Phosphorylation of Dab1 is detected by immunoprecipitation (IP) of total Dab1 followed by western blot (WB) anti-phosphotyrosines. Negative control of IP and basal levels of Dab1 phosphorylation are shown respectively in lanes 1 and 2. Mock sample does not induce changes in the basal levels of Dab1 phosphorylation (Lane 3). Reelin supernatants induce a high increase in the phosphorylation of Dab1 (Lane 4). Purified Reelin is also functional (Lane 5) and maintains its activity after nitrogen freezing and lyophilization (Lanes 6 and 7). ( b ) Densitometric analysis of phosphorylated Dab1 WB images shows a 6–8-fold increase upon Reelin treatment in one to three independent experiments ( n =3 for lanes 2–4; n =2 for lanes 1,5 and 6 and n =1 for lane 7). Full-size blots can be found in Supplementary Fig. 1 . Data are represented as mean±s.e.m. Full size image To characterize whether Reelin modifies the kinetics of Aβ 42 aggregation into amyloid fibrils, a freshly isolated Aβ 42 preparation (24 μM), which contained monomeric Aβ 42 in rapid equilibrium with low-molecular weight (LMW) oligomers, was allowed to aggregate in low-salinity conditions in the presence or absence of either purified Reelin or equivalent volumes of Mock control. The following mixtures were run in parallel: Aβ 42 ; Aβ 42 :Reelin (Aβ 42 /Rln) in a ratio 6:1 w / w (that is, Aβ 42 108 ng μl −1 and Reelin 18 ng μl −1 ) and Aβ 42 :Mock control (Aβ 42 /Mock). In addition, Reelin (Rln) and Mock preparations without the addition of Aβ 42 were also tested. To monitor fibril formation, both thioflavin-T (ThT) fluorescence assay and transmission electron microscopy (TEM) were carried out every 24 h. In the absence of Reelin (that is, Aβ 42 and Aβ 42 /Mock samples) a time-dependent increase in ThT fluorescence emission was observed from day 7 onwards ( Fig. 3a ). The lag phase of fibril formation was calculated by adjusting a sigmoidal curve to the experimental data (that is, 8.3 days for Aβ 42 and 7.9 days for Aβ 42 /Mock). The ThT-binding assay of Aβ 42 /Rln samples showed a consistent slowdown in the kinetics of the process, with a 2.5-day delay in the start of fibril formation ( Fig. 3a ) and an estimated lag-phase duration of 10.9 days. In agreement with ThT data, TEM images obtained during the lag phases showed amorphous deposits without fibrils ( Fig. 3b ). At day 9, isolated fibril-like structures started to appear in Aβ 42 and Aβ 42 /Mock samples, with fully mature fibrils being observed from day 11 onwards, coincident with maximal ThT emission fluorescence ( Fig. 3b , upper panels). As expected from the ThT data, TEM of Aβ 42 /Rln samples showed a 2-day delay in the appearance of fibrils. Short isolated fibrils appeared at day 11 and fully mature fibrils from day 13 onwards ( Fig. 3b , bottom panels). The delay in Aβ 42 aggregation induced by Reelin was corroborated in a different kinetic and saline concentration experiment, which also showed a dose-dependent Reelin effect ( Fig. 4 ). 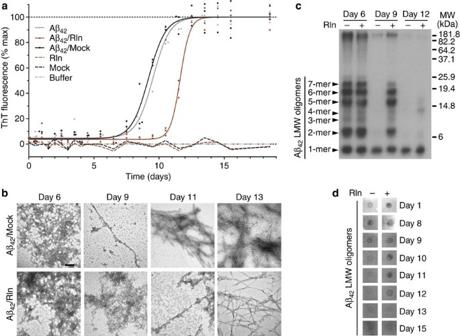Figure 3: Reelin delays the kinetics of Aβ42fibril formation. (a) Time-course quantification of amyloid fibril content in Aβ42(24 μM) preparations by the Thioflavin-T (ThT)-binding assay. When Reelin is incubated with Aβ42(Aβ42/Rln sample 6:1 (w/w)), it induces a 2.5-day delay in the appearance of fibrils. (b) TEM micrographs obtained during the time-course of aggregation showing that mature fibril structures appear with a 2-day delay when Reelin is present (lower panels). (c) Western blot detection of Aβ peptides after PICUP at various time-points during Aβ42aggregation in the presence or absence of Reelin. Reelin extends the time-window in which LMW oligomeric species of 2- to 7-mer are present. (d) A11 oligomer-specific immunoreactivity against HMW Aβ oligomeric species in the presence and absence of Reelin. Reelin extends the time-window in which HMW oligomeric species of >40 KDa are present. Scale bar: (b), 100 nm. Figure 3: Reelin delays the kinetics of Aβ 42 fibril formation. ( a ) Time-course quantification of amyloid fibril content in Aβ 42 (24 μM) preparations by the Thioflavin-T (ThT)-binding assay. When Reelin is incubated with Aβ 42 (Aβ 42 /Rln sample 6:1 ( w / w )), it induces a 2.5-day delay in the appearance of fibrils. ( b ) TEM micrographs obtained during the time-course of aggregation showing that mature fibril structures appear with a 2-day delay when Reelin is present (lower panels). ( c ) Western blot detection of Aβ peptides after PICUP at various time-points during Aβ 42 aggregation in the presence or absence of Reelin. Reelin extends the time-window in which LMW oligomeric species of 2- to 7-mer are present. ( d ) A11 oligomer-specific immunoreactivity against HMW Aβ oligomeric species in the presence and absence of Reelin. Reelin extends the time-window in which HMW oligomeric species of >40 KDa are present. Scale bar: ( b ), 100 nm. 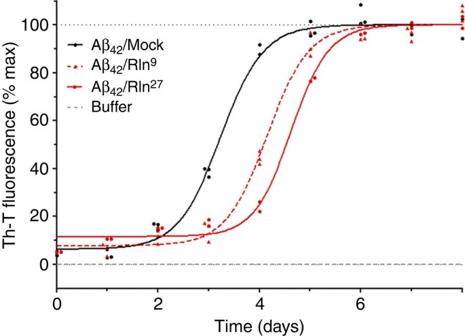Figure 4: Reelin delays Aβ42fibril formation in a concentration-dependent manner. Time-course of amyloid fibrillization detected by Thioflavin-T binding assay in Aβ42(24 μM) preparations and 17 mM NaCl, using two Reelin concentrations (9 and 27 ng μl−1, corresponding to an Aβ42:Reelin ratio of 12:1 and 4:1 respectively). A delay proportional to Reelin concentration is produced. The black curve represents Aβ42/Mock aggregation (lag-phase duration: 1.23 days); the red dashed curve represents Aβ42/Rln 9 ng μl−1(lag-phase duration: 2.15 days); the red continuous curve represents Aβ42/Rln 27 ng μl−1(lag-phase duration: 2.63 days). Full size image Figure 4: Reelin delays Aβ 42 fibril formation in a concentration-dependent manner. Time-course of amyloid fibrillization detected by Thioflavin-T binding assay in Aβ 42 (24 μM) preparations and 17 mM NaCl, using two Reelin concentrations (9 and 27 ng μl −1 , corresponding to an Aβ 42 :Reelin ratio of 12:1 and 4:1 respectively). A delay proportional to Reelin concentration is produced. The black curve represents Aβ 42 /Mock aggregation (lag-phase duration: 1.23 days); the red dashed curve represents Aβ 42 /Rln 9 ng μl −1 (lag-phase duration: 2.15 days); the red continuous curve represents Aβ 42 /Rln 27 ng μl −1 (lag-phase duration: 2.63 days). Full size image To gain insight into the molecular mechanisms of the Reelin-induced delay in fibril formation, we studied the nature of the Aβ 42 oligomeric species formed before fibril formation. We analysed the distribution of LMW Aβ 42 oligomers (from dimers to heptamers) using Photo-Induced Crosslink of Unmodified Proteins (PICUP) [29] , followed by western blotting against Aβ peptide. Before the appearance of fibrils, the distribution of LMW oligomeric species did not vary between Aβ 42 /Mock and Aβ 42 /Rln samples ( Fig. 3c , lanes 1 and 2). In contrast, during the 2-day delay in fibril formation exerted by Reelin, LMW oligomers disappeared from the Aβ 42 /Mock samples, but not from Aβ 42 /Rln samples ( Fig. 3c , lanes 3 and 4). LMW oligomers were no longer detected when fibrils were present in Aβ 42 /Mock and Aβ 42 /Rln samples ( Fig. 3c , lanes 5 and 6). The effect of Reelin on the formation of high-molecular weight (HMW) soluble oligomers was also studied by dot blot analysis with the A11 antibody [30] . Our results again showed a 2-day delay in the A11-specific signal loss during aggregation in the Aβ 42 /Rln sample, as compared with the Aβ 42 /Mock control ( Fig. 3d ). These results indicate that Reelin delays the aggregation of Aβ 42 into fibrils in vitro and that it extends the lifetime of LMW and HMW oligomeric species. Reelin interacts with Aβ 42 and is sequestered by fibrils To examine the possible interaction between Reelin and soluble Aβ 42 species, we performed immunoprecipitation assays of Aβ 42 /Rln samples (obtained at pre-fibrillar stages of aggregation). Western blot analysis of anti-Aβ and anti-Reelin immunoprecipitated samples revealed a specific interaction between Reelin and soluble Aβ 42 species ( Fig. 5a ). 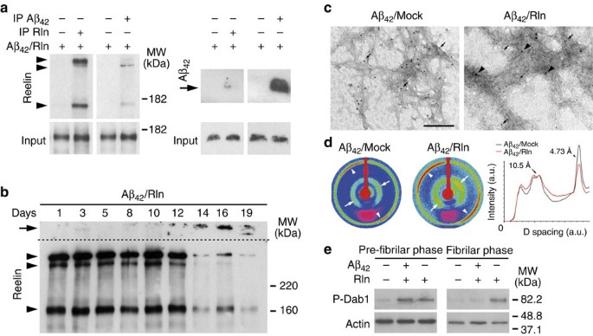Figure 5: Reelin interacts with aggregating Aβ42until it becomes trapped in fibrils. (a) Aβ42and Reelin immunoprecipitation on pre-fibrillar Aβ42/Rln, followed by western blot against either Reelin (arrowheads; left panels) or Aβ (arrow; right panels). Negative controls of non-immunoprecipitated samples are shown in lanes 1, 3, 5 and 7 (upper panels). Lanes 2 and 8 show the positive controls of immunoprecipitated Reelin and Aβ42respectively (upper panels). Reelin and Aβ co-immunoprecipitate, as shown in lanes 4 and 6, indicating a specific interaction. Lower panels show input samples for Reelin (180 kDa band; left panels) and Aβ42(right panels) before immunoprecipitation. (b) Western blot of Reelin during the time-course of Aβ42/Rln aggregation showing a decrease in soluble Reelin (arrowheads), coinciding with the time-point when Aβ42fibrils start appearing. A Reelin-specific signal appears at the bottom of the well, indicating the presence of this protein in insoluble debris (arrow). (c) Transmission electron micrographs of double immunogold labelling of Aβ (12-nm particles; arrows) and Reelin (18-nm particles; arrowheads). Reelin-specific signal is detected colocalizing with fibrils. (d) X-ray fibril diffraction pattern for aligned fibrils showing the two characteristic reflection arcs on the equatorial (parallel with the fibril axis at 4.73 Å (arrowheads) and a signal on the meridional at 10.5 Å (arrows). Diffraction signal intensity is pseudo-colored in ImageJ software using spectrum LUT. One-dimensional azimuthal plots showing intensity of diffractions as a function of D-spacing indicates that, in the presence of Reelin, the structure of the fibrils is conserved. (e) Reelin activity assessed as the capacity to induce phosphorylation on Dab1 protein after 15 min treatment of neuronal primary cultures. Reelin induces phosphorylation of Dab1 even in the presence of Aβ42and before fibril formation (pre-fibrillar phase) but not after the formation of fibrils (fibrillar phase). Reelin without Aβ42under the same conditions retains its activity throughout the timescale of the experiment. Full-size blots can be found inSupplementary Figs 2 and 3. Scale bar: (c), 200 nm. Figure 5: Reelin interacts with aggregating Aβ 42 until it becomes trapped in fibrils. ( a ) Aβ 42 and Reelin immunoprecipitation on pre-fibrillar Aβ 42 /Rln, followed by western blot against either Reelin (arrowheads; left panels) or Aβ (arrow; right panels). Negative controls of non-immunoprecipitated samples are shown in lanes 1, 3, 5 and 7 (upper panels). Lanes 2 and 8 show the positive controls of immunoprecipitated Reelin and Aβ 42 respectively (upper panels). Reelin and Aβ co-immunoprecipitate, as shown in lanes 4 and 6, indicating a specific interaction. Lower panels show input samples for Reelin (180 kDa band; left panels) and Aβ 42 (right panels) before immunoprecipitation. ( b ) Western blot of Reelin during the time-course of Aβ 42 /Rln aggregation showing a decrease in soluble Reelin (arrowheads), coinciding with the time-point when Aβ 42 fibrils start appearing. A Reelin-specific signal appears at the bottom of the well, indicating the presence of this protein in insoluble debris (arrow). ( c ) Transmission electron micrographs of double immunogold labelling of Aβ (12-nm particles; arrows) and Reelin (18-nm particles; arrowheads). Reelin-specific signal is detected colocalizing with fibrils. ( d ) X-ray fibril diffraction pattern for aligned fibrils showing the two characteristic reflection arcs on the equatorial (parallel with the fibril axis at 4.73 Å (arrowheads) and a signal on the meridional at 10.5 Å (arrows). Diffraction signal intensity is pseudo-colored in ImageJ software using spectrum LUT. One-dimensional azimuthal plots showing intensity of diffractions as a function of D-spacing indicates that, in the presence of Reelin, the structure of the fibrils is conserved. ( e ) Reelin activity assessed as the capacity to induce phosphorylation on Dab1 protein after 15 min treatment of neuronal primary cultures. Reelin induces phosphorylation of Dab1 even in the presence of Aβ 42 and before fibril formation (pre-fibrillar phase) but not after the formation of fibrils (fibrillar phase). Reelin without Aβ 42 under the same conditions retains its activity throughout the timescale of the experiment. Full-size blots can be found in Supplementary Figs 2 and 3 . Scale bar: ( c ), 200 nm. Full size image We next analysed the distribution of Reelin in Aβ 42 /Rln samples taken at the fibrillar stage of aggregation, when insoluble Aβ 42 fibrils are formed. Western blot analysis of Aβ 42 /Rln aliquots taken during aggregation revealed that concomitantly with the start of fibril formation, Reelin bands disappear from their expected MW and appear at the well-bottom of the SDS-PAGE gel ( Fig. 5b , lanes 7–9). This finding suggests that Reelin is sequestered into the assembling amyloid fibrils. As a further indication of the Reelin–Aβ 42 –fibril interaction, Aβ 42 /Rln fibrils assembled in vitro were subjected to double immunogold labelling for Reelin and Aβ 42 . Electron micrographs revealed the colocalization of Reelin and Aβ 42 in the aggregated fibrils in vitro ( Fig. 5c ) Taken together, our experiments with purified Reelin and Aβ 42 show a direct interaction between Reelin and Aβ 42 at early pre-fibrillar stages of amyloid aggregation. Moreover, in the fibrillar stage of amyloid aggregation, our data support the interaction of Reelin and Aβ 42 fibrils, which occurs independently of additional partners that may be present in the senile plaques in vivo . To analyse whether the presence of Reelin in Aβ 42 fibrils affects their structural properties, we examined dried fibrils by X-ray diffraction analysis. Aβ 42 /Mock and Aβ 42 /Rln fibrils showed the two characteristic perpendicular reflection arcs at equatorial (4.73 Å) and meridional (10.5 Å) axes, corresponding to the fibrillar cross-beta structure of aligned fibrils ( Fig. 5d ). This observation indicates that Reelin does not modify the fibrillar structure, and suggests that it interacts with Aβ 42 along the surface of the fibril. Next, we analysed the biological activity of Reelin by measuring the phosphorylation levels of the Reelin transducer Dab1 in primary neuronal forebrain cultures treated with purified Reelin or with Aβ 42 /Mock and Aβ 42 /Rln samples taken at the pre-fibrillar or fibrillar stages. Samples that were not treated with Reelin showed basal levels of Dab1 phosphorylation ( Fig. 5e , lanes 1 and 4). Aβ 42 /Rln samples induced the phosphorylation of Dab1 at the pre-fibrillar stage, but not at the fibrillar stage ( Fig. 5e , lanes 2 and 5), while Reelin without Aβ 42 retained its biological activity throughout the experiment ( Fig. 5e , lanes 3 and 6). All together, these data indicate that, by interacting with soluble Aβ 42 species, Reelin delays Aβ 42 fibril formation until it becomes trapped in the amyloid fibrils, when it loses its biological signalling activity. Reelin reduces amyloid deposits in AD mice To evaluate the in vivo impact of Reelin on Aβ peptide aggregation we crossed transgenic mice overexpressing Reelin under the control of the CAMKIIα promoter (TgRln) [13] with AD mice carrying the hAPP Swe/Ind mutation (J20) [26] , (TgRln/J20). We measured amyloid plaque load in the hippocampus by quantifying the area occupied by plaques at 4, 8 and 12 months of age. At the onset of plaque deposition (4 months) a very small number of plaques were present in J20 and TgRln/J20 mice with no significant differences between groups. At a later stage (8 months) plaque load was still minimal in J20 and TgRln/J20 groups ( Fig. 6a,b ). At 12 months of age, the percentage of area occupied by plaques in the hippocampus was significantly lower in TgRln/J20 than in J20 mice ( Fig. 6a,b ). The same plaque reduction held true in TgRln/J20 mice in the entorhinal cortex ( Fig. 6a,b ). Taken together, our results indicate a similar onset of plaque appearance in both genotypes, with TgRln/J20 mice showing a reduced number of deposits at 12 months of age. These results are consistent with our previous in vitro observations of a Reelin-dependent delay in the formation of Aβ 42 fibrils. 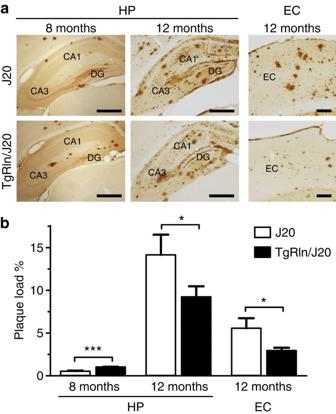Figure 6: Reelin overexpression reduces plaque content in 12-month-old J20 mice. (a) Immunohistochemical detection of amyloid plaques (3D6 antibody) in 8- and 12-month-old hippocampal sections and 12-month-old entorhinal cortex sections from J20 and TgRln/J20 mice. (b) Plaque load in the hippocampus of 8-month-old TgRln/J20 animals is higher than in J20 mice. The area occupied by plaques in 12-month-old TgRln/J20 animals is markedly reduced both in the hippocampus and entorhinal cortex.n=3–5 animals per group, 6–8 sections per animal. Scale bars: (a) left, middle:, 500 μm; right, 200 μm. HP, hippocampus; EC; entorhinal cortex; CA1–CA3, hippocampal regions; DG, dentate gyrus. Data are represented as mean±s.e.m.; *P<0.05; ***P<0.001; Student’st-test. Figure 6: Reelin overexpression reduces plaque content in 12-month-old J20 mice. ( a ) Immunohistochemical detection of amyloid plaques (3D6 antibody) in 8- and 12-month-old hippocampal sections and 12-month-old entorhinal cortex sections from J20 and TgRln/J20 mice. ( b ) Plaque load in the hippocampus of 8-month-old TgRln/J20 animals is higher than in J20 mice. The area occupied by plaques in 12-month-old TgRln/J20 animals is markedly reduced both in the hippocampus and entorhinal cortex. n =3–5 animals per group, 6–8 sections per animal. Scale bars: ( a ) left, middle:, 500 μm; right, 200 μm. HP, hippocampus; EC; entorhinal cortex; CA1–CA3, hippocampal regions; DG, dentate gyrus. Data are represented as mean±s.e.m. ; * P <0.05; *** P <0.001; Student’s t -test. Full size image Reelin reduces Aβ 42 oligomer toxicity and rescues spine loss Soluble Aβ 42 oligomers are considered to be the pathogenic molecular form of Aβ peptide in AD [4] . To test how Reelin affects Aβ 42 oligomer-induced cytotoxicity, we used a standard preparation of soluble Aβ oligomers: Aβ-derived diffusible ligands (ADDLs) [6] . We first corroborated the interaction of Reelin and Aβ 42 ADDLs ( Fig. 7 ). Then, we treated primary hippocampal neuronal cultures for 24 h with ADDLs, plus either Reelin or Mock purified supernatants. Neuronal damage was assessed by the analysis of propidium iodide (PI) nuclear staining. Exposure of the cultures to ADDLs (5 or 10 μM) plus Mock caused an increase in PI nuclear staining, as compared with treatments with vehicle (100% survival) ( Fig. 8a,b ). Reelin increased neuronal survival after treatment with 5–10 μM ADDLs ( Fig. 8b ). 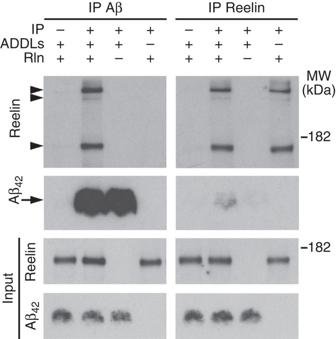Figure 7: Reelin interacts with Aβ42in the form of ADDLs. Aβ42and Reelin immunoprecipitation (IP) after 1-h incubation of purified Reelin with ADDLs. IP was followed by western blot (WB) against either Reelin or Aβ, as indicated. Negative controls of non-immunoprecipitated samples are shown in lanes 1 and 5 (upper panels). Reelin and Aβ are co-immunoprecipitated, as shown in lanes 2 and 6, indicating a specific interaction. Lower panels show input samples before immunoprecipitation, as indicated. Full-size blots can be found inSupplementary Fig. 4. Figure 7: Reelin interacts with Aβ 42 in the form of ADDLs. Aβ 42 and Reelin immunoprecipitation (IP) after 1-h incubation of purified Reelin with ADDLs. IP was followed by western blot (WB) against either Reelin or Aβ, as indicated. Negative controls of non-immunoprecipitated samples are shown in lanes 1 and 5 (upper panels). Reelin and Aβ are co-immunoprecipitated, as shown in lanes 2 and 6, indicating a specific interaction. Lower panels show input samples before immunoprecipitation, as indicated. Full-size blots can be found in Supplementary Fig. 4 . 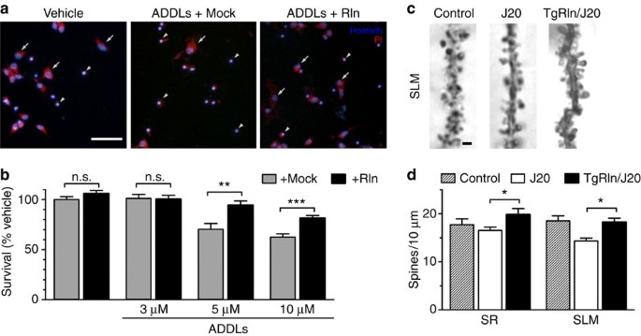Figure 8: Reelin ameliorates the toxicity of ADDLs and reverses dendritic spine loss in J20 mice. (a) Representative images from neuronal primary cultures treated for 24 h and labelled with PI and Hoechst 33342. Dying neurons show double-labelled picnotic nuclei (arrowheads). Healthy cells are indicated by arrows. Treatments were performed with 5 μM of ADDLs with Reelin (Rln) added at 5 ng μl−1, or equivalent volumes of Mock. (b) Quantification of cell survival after a 24-h treatment showing that the toxicity of ADDLs at 5–10 μM is significantly reduced by Rln.n=15–40 microscopy fields per condition from four independent experiments. (c) Micrographs illustrating representative stratum lacunosum moleculare dendrites from control, J20 and TgRln/J20 animals after Golgi staining. (d) Quantification of the density of dendritic spines showing that spine reduction in J20 mice is rescued in TgRln/J20 animals.n=3 mice per genotype, 20–35 neurons. Scale bars: (a), 200 μm; (c), 1 μm. SR, stratum radiatum; SLM, stratum lacunosum moleculare. Data are represented as mean±s.e.m.; n.s. (non-significant);P>0.05; *P<0.05; **P<0.01; ***P<0.001; Student’st-test. Full size image Figure 8: Reelin ameliorates the toxicity of ADDLs and reverses dendritic spine loss in J20 mice. ( a ) Representative images from neuronal primary cultures treated for 24 h and labelled with PI and Hoechst 33342. Dying neurons show double-labelled picnotic nuclei (arrowheads). Healthy cells are indicated by arrows. Treatments were performed with 5 μM of ADDLs with Reelin (Rln) added at 5 ng μl −1 , or equivalent volumes of Mock. ( b ) Quantification of cell survival after a 24-h treatment showing that the toxicity of ADDLs at 5–10 μM is significantly reduced by Rln. n =15–40 microscopy fields per condition from four independent experiments. ( c ) Micrographs illustrating representative stratum lacunosum moleculare dendrites from control, J20 and TgRln/J20 animals after Golgi staining. ( d ) Quantification of the density of dendritic spines showing that spine reduction in J20 mice is rescued in TgRln/J20 animals. n =3 mice per genotype, 20–35 neurons. Scale bars: ( a ), 200 μm; ( c ), 1 μm. SR, stratum radiatum; SLM, stratum lacunosum moleculare. Data are represented as mean±s.e.m. ; n.s. (non-significant); P >0.05; * P <0.05; ** P <0.01; *** P <0.001; Student’s t -test. Full size image Aβ oligomers are reported to mediate synaptic dysfunction [31] . We next sought to determine whether Reelin overexpression protects against the synaptopathological features observed in J20 mice, in which a decreased number of synaptic contacts and dendritic spines has been described [32] . Eight-month-old mice were processed for Golgi staining, and dendritic spines were counted in secondary pyramidal cell dendrites (CA1 region) in the stratum radiatum and stratum lacunosum moleculare ( Fig. 8c ). In both layers, the dendritic spine densities were similar in TgRln/J20 and control mice, and significantly higher in TgRln/J20 compared with J20 animals ( Fig. 8d ), indicating that Reelin overexpression significantly rescued the loss of dendritic spines in this AD model. Taken together, our data indicate that, by interacting with Aβ species, Reelin protects against both Aβ-induced neurotoxicity and dendritic spine loss. Reelin rescues cognitive impairment in AD and aged mice As a reduced number of synaptic contacts in AD mice correlates with cognitive deficits [33] , we next analysed whether Reelin overexpression could improve cognitive performance in TgRln/J20 mice. J20 animals show cognitive impairment even before the appearance of amyloid deposits, including deficits in the novel object recognition (NOR) task [34] . We tested the effect of Reelin overexpression on these behavioural alterations by performing the NOR task in 4–5 and 8–10-month-old littermate mice (genotypes: control, TgRln, J20 and TgRln/J20). Control and TgRln animals, from both age groups, spent a significantly higher proportion of time exploring the new object versus a familiar one than J20 animals, reflected in a higher discrimination index. This result indicates cognitive deficits in the J20 animals, as previously described [34] . Interestingly, this cognitive deficit was not present in TgRln/J20 animals, which presented a discrimination index similar to control animals, at both 4–5 and 8–10 months ( Fig. 9a ). These data indicate that Reelin overexpression leads to a reversion of the recognition memory deficits observed in J20 mice up to 8–10 months of age. 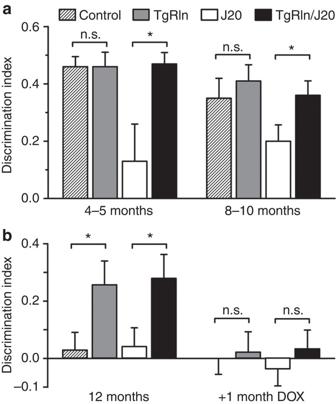Figure 9: Reelin overexpression reverses behavioural phenotypes in J20 AD mice. (a) The NOR task was performed on littermates with different genotypes (WT, TgRln, J20 and TgRln/J20) at the ages of 4–5 and 8–10 months. At both time-points tested, the performance of J20/TgRln animals was significantly better than that of J20 mice. (b) Animals were also assayed at the age of 12 months, and, immediately after the NOR task, the same group of animals was treated with DOX-diet (200 mg per kg) for 1 month and tested again for NOR. Reelin overexpression prevented age-related cognitive decline in both J20 and in non-J20 animals. This improved performance was dependent on Reelin overexpression as DOX treatment completely abolished discrimination.n=8–12 mice per group. Data are represented as mean±s.e.m.; n.s. (non-significant);P>0.05; *P<0.05; Student’st-test. Figure 9: Reelin overexpression reverses behavioural phenotypes in J20 AD mice. ( a ) The NOR task was performed on littermates with different genotypes (WT, TgRln, J20 and TgRln/J20) at the ages of 4–5 and 8–10 months. At both time-points tested, the performance of J20/TgRln animals was significantly better than that of J20 mice. ( b ) Animals were also assayed at the age of 12 months, and, immediately after the NOR task, the same group of animals was treated with DOX-diet (200 mg per kg) for 1 month and tested again for NOR. Reelin overexpression prevented age-related cognitive decline in both J20 and in non-J20 animals. This improved performance was dependent on Reelin overexpression as DOX treatment completely abolished discrimination. n =8–12 mice per group. Data are represented as mean±s.e.m. ; n.s. (non-significant); P >0.05; * P <0.05; Student’s t -test. Full size image In 12-month-old mice, the performance of control mice did not differ from that of J20 animals ( Fig. 9b ), consistent with an age-dependent cognitive decline [35] . In contrast, the discrimination index of TgRln mice aged 12 months was significantly higher than that of the control group. Interestingly, 12-month-old TgRln/J20 animals performed better than controls and J20 mice, thereby retaining recognition capacity levels similar to those shown by TgRln mice, despite the abnormal Aβ production ( Fig. 9b ). To ascertain whether these protective behavioural effects were specifically caused by Reelin, the same groups of animals were tested 1 month after the administration of doxycycline, used to stop Reelin transgene expression [13] . Upon transgene inactivation, the discrimination index diminished to zero in both TgRln and TgRln/J20 mice, thereby indicating a complete loss of long-lasting Reelin-dependent protection after 1 month of depletion ( Fig. 9b ). Taken together, our data show that Reelin overexpression ameliorates age-dependent cognitive decline in control animals. Moreover, Reelin overexpression is sufficient to protect and fully recover the recognition memory impairment caused by Aβ production in J20 mice. Functional links between the Reelin pathway and AD include molecular cross-talk between the Reelin signalling pathway and both APP processing and Tau phosphorylation [15] , [16] , altered expression of Reelin in AD brains [18] , [19] , [20] , [21] , [22] , the presence of Reelin in amyloid plaques [14] and genetic RLN variants linked to AD [23] , [24] . However, the contribution of Reelin to AD pathogenesis and progression is not yet understood [36] . Here we addressed the relationships between Reelin and Aβ aggregation and show that, both in vitro and in vivo , Reelin modifies the kinetics of Aβ 42 aggregation, delaying amyloid fibril formation. Furthermore, Reelin interacts with Aβ 42 soluble species, reduces their toxicity and rescues the Aβ 42 -induced loss of dendritic spines in vivo . Finally, we show that Reelin overexpression rescues the recognition memory deficits during normal ageing as well as in J20 AD mice. Taken together, these results highlight the potential of Reelin as a neuroprotective tool and cognitive enhancer during normal ageing and AD pathogenesis, as it has the capacity to overcome the deficits associated with Aβ deposition. The kinetics of Aβ 42 fibril formation is highly dependent on Aβ 42 concentration, temperature and salinity. Our data show slower kinetics than that reported in other studies [37] , [38] due to the conditions of low salinity and temperature used, which were initially selected to analyse the early pre-fibrillar stage of aggregation. However, using distinct salt and Reelin concentrations, here we demonstrate that Reelin slows down the kinetics of Aβ 42 fibril formation and extends the lifespan of Aβ 42 oligomers. Moreover, the present study shows for the first time a direct interaction between Reelin and soluble Aβ 42 . Importantly, our experimental evidence demonstrates that Reelin protects against Aβ 42 oligomer-induced toxicity, including neuronal degeneration triggered by ADDLs in cultured neurons and Aβ-stimulated dendritic spine loss in J20 AD mice. Both pathological processes are believed to be mediated mainly by Aβ 42 oligomeric species [5] . A full understanding of the molecular mechanisms by which Reelin extends the lifetime and overcomes the toxicity of Aβ 42 oligomers clearly requires further research. However, one hypothesis is that the interaction of Reelin with soluble Aβ 42 may induce conformational and structural changes in Aβ 42 oligomers that affect their biological properties, including aggregation and toxicity. In turn, the Aβ 42 oligomer–Reelin interaction would result in delayed fibril formation and reduced amyloid plaque load in TgRln/J20 mice. We also demonstrate that Reelin interacts with amyloid fibrils. The observation that Reelin does not modify the structural properties of the fibrils suggests that Reelin interacts with Aβ 42 fibrils in a non-regular manner, most likely at their surface. The interaction of Reelin with amyloid fibrils could stabilize the latter, preventing Aβ molecules from recycling through fibril ends [39] . Moreover, this interaction could also affect secondary nucleation processes, a newly proposed mechanism associated with the formation of Aβ oligomers from Aβ monomers catalysed by the fibril surface [37] . Thus, the interaction of Reelin with the Aβ 42 fibrils is likely to be responsible for overcoming the toxic mechanisms associated with amyloid fibrils [40] . This study also shows that Reelin overexpression in J20 mice is sufficient to achieve functional recovery of behavioural deficits, as shown by the NOR task. An important difference between the in vivo and in vitro results reported here is that in our transgenic mice neuroprotection occurs under a context of continuous production of both Reelin and Aβ 42 . Interestingly, Reelin fully rescued spatial, recognition memory deficits in J20 mice throughout life, preventing the appearance of AD-related cognitive impairment even in ageing J20 mice, after continuous production of Aβ 42. Finally, our transgene switch-off experiments not only demonstrate the specificity of the observed phenotypes for the Reelin pathway but also that this neuroprotection depends on the acute production and activation of the Reelin cascade. In addition, here we show that the trapping of Reelin into Aβ 42 fibrils causes the loss of Reelin signalling itself. In the adult brain, the Reelin pathway has been shown to favour α-processing of APP, decrease GSK3β activity and Tau phosphorylation, potentiate glutamatergic neurotransmission, LTP and structural synaptic plasticity, and to positively regulate adult neurogenesis in the hippocampus [13] , [15] , [16] , [41] , [42] . These processes are necessary for correct neuronal physiology and cognitive adult functions and are impaired in AD. We thus propose that the Reelin cascade is a key ‘homoeostatic’ pathway that regulates numerous aspects of normal adult brain function and whose dysfunction may contribute to the pathological and cognitive traits typical of AD. This vision is in agreement with the view that Reelin depletion in the temporal lobe is one of the early events in AD pathogenesis [22] and with studies reporting that Reelin haploinsufficiency in AD mice results in accelerated AD-like pathology [25] , [43] . In summary, our data support a model ( Fig. 10 ) in which the Reelin pathway exerts beneficial effects on both AD pathology and cognition by at least two complementary mechanisms. In addition to extracellular Reelin delaying amyloid fibril formation and reducing neurotoxicity by interacting with Aβ 42 soluble species and fibrils, the activation of the Reelin cascade itself would potentiate adult plasticity events, including synaptic plasticity and adult neurogenesis, and lead to decreased GSK3β activity and Tau phosphorylation. On the basis of our findings in transgenic mice, we propose that the acute activation of the Reelin pathway represents a new therapeutic strategy for ameliorating the cognitive decline associated with normal ageing and the deficits characteristic of AD pathology. 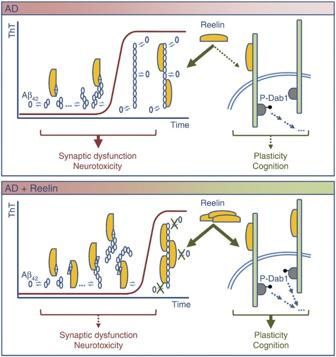Figure 10: Summary scheme illustrating the involvement of Reelin in Alzheimer’s disease. In AD (upper panel), high levels of neurotoxic soluble Aβ oligomers induce a wide range of alterations, including synaptic dysfunction. Reelin interacts with soluble Aβ species and gets trapped in amyloid fibrils, where it loses its functionality, resulting in a downregulation of the Reelin signalling pathway. Increased Reelin levels in the context of AD (lower panel), possibly through enhanced Aβ-Reelin interaction, lead to delayed fibril formation, reduced plaque load and decreased Aβ toxicity, with a recovery of synaptic loss and cognitive functions. Additionally, increased levels of functional Reelin might restore its downstream signalling pathway, further exerting neuroprotection. By these two complementary mechanisms, increased Reelin levels in AD overcome Aβ-mediated toxicity and cognitive deficits. These observations point to the Reelin pathway as a new therapeutic target for the treatment of AD. Figure 10: Summary scheme illustrating the involvement of Reelin in Alzheimer’s disease. In AD (upper panel), high levels of neurotoxic soluble Aβ oligomers induce a wide range of alterations, including synaptic dysfunction. Reelin interacts with soluble Aβ species and gets trapped in amyloid fibrils, where it loses its functionality, resulting in a downregulation of the Reelin signalling pathway. Increased Reelin levels in the context of AD (lower panel), possibly through enhanced Aβ-Reelin interaction, lead to delayed fibril formation, reduced plaque load and decreased Aβ toxicity, with a recovery of synaptic loss and cognitive functions. Additionally, increased levels of functional Reelin might restore its downstream signalling pathway, further exerting neuroprotection. By these two complementary mechanisms, increased Reelin levels in AD overcome Aβ-mediated toxicity and cognitive deficits. These observations point to the Reelin pathway as a new therapeutic target for the treatment of AD. Full size image Animals TgRln (Tg1/Tg2) is a conditional regulated transgenic line that overexpresses Reelin under the control of the calcium–calmodulin-dependent kinase II α promoter (pCaMKIIα) [13] . Line J20 produces hAPP with the Swedish (KM670/671NL) and Indiana (V717F) mutations (hAPP Swe/Ind ) under the control of platelet-derived growth factor promoter [26] . J20 was purchased from Jackson. All the transgenic animals used in this study were kept in hemizygosis for each transgene. Mice were bred in the animal research facilities at the Barcelona Science Park and at the University of Barcelona. The NOR task was performed at the Barcelona Biomedical Research Park. Animals were provided with food and water ad libitum and maintained in a temperature-controlled environment in a 12/12 h light-dark cycle. For doxycycline treatment, 12-month-old adult male mice were fed ad libitum with doxycycline-containing feed (Bio-Serv, 200 mg per kg). All the experiments involving animals were performed in accordance with the European Community Council directive and the National Institute of Health guidelines for the care and use of laboratory animals. Experiments were also approved by the local ethical committees. Antibodies and reagents Mouse monoclonal anti-Aβ amino acids 1–5 (clone 3D6) were provided by Elan Pharmaceuticals and used for histological plaque staining (1:500). The commercial primary antibodies used were: anti-Reelin (clone G10, MAB5364, Millipore, 1:1,000), anti-Dab1 (AB5840, Millipore, 1:1,000), anti-Aβ (clone 6E10, SIG-39320, Covance, 1:1,000), anti-phosphotyrosines (clone 4G10, 05-521, Millipore, 1:1,000), anti-β-Tubulin (clone AA2, 05-661, Millipore, 1:1,000) and anti-actin (MAB1501, Millipore, 1:100,000) for western blot; anti-Dab1 (U100P, ExAlpha, 3 μg per sample), anti-Aβ (6E10, 2 μg per sample) and anti-Reelin (G10, 2 μg per sample) for immunoprecipitation; anti-oligomers (A11, AHB0052, Invitrogen, 3 μg ml −1 ) for dot blot; and anti-Aβ 40/42 (AB5076, Chemicon, 1:25) and anti-Reelin (G10, 1:25) for immunogold labelling. The secondary antibodies used were the following: HRP-labelled anti-mouse (P447-01, Vector, 1:2,000) and anti-rabbit (P217-02, Vector, 1:2,000) for western blot; biotinylated anti-mouse (BA2000, Vector, 1:200) for histological plaque staining; and colloidal gold-coated anti-mouse (18 nm, 115-215-146, Jackson, 1:30) and anti-rabbit (12 nm, 114-205-144, Jackson, 1:30) for immunogold labelling. Streptavidin–biotinylated/HRP complex, and Protein A and Protein G Sepharose 4 Fast Flow were from GE Healthcare. F(ab′)2 fragment anti-mouse IgG was from Jackson. Thioflavin-T (ThT), ammonium persulfate (APS), tris(bipyridine)ruthenium(II) chloride (Ru(bpy) 3 2+ ), diaminobenzidine reagent (DAB), hydrogen peroxide (H 2 O 2 ), Hoechst 33342 and PI were from Sigma. Reelin production and purification Reelin supernatants were prepared from 293T cells stably transfected with full-length Reelin clone pCrl (the cells were a gift from the Frotscher laboratory) [44] and cultured with OPTI-MEM medium (GIBCO). The collected Reelin supernatants were washed with double the initial volume of 10 mM phosphate buffer (PB)/30 mM NaCl (pH 7.4) and concentrated 10-fold using ultrafiltration Vivaflow 50 filters (Sartorius; 100 kDa MWCO), previously blocked with 1% BSA. Concentrated supernatants were subjected to anion exchange chromatography performed with a HiTrap IEX ANX column (GE Healthcare), mobile phase NaCl 30 mM/PB 10 mM (pH 7.6), at a flow rate of 2 ml min −1 . Sample fractionation was performed by a five-step gradient elution, increasing NaCl concentration from 30 mM up to 150, 250, 350, 650 and 1,000 mM in an FPLC system. Reelin-containing fractions eluting at 350 mM NaCl were collected and concentrated 10-fold using Vivaspin filters (Sartorius; 100 kDa MWCO), previously blocked with 1% BSA. Concentrated samples were loaded onto a 25 ml pre-packed Superose 6 10/300 size exclusion column (GE Healthcare), previously equilibrated with 10 mM PB/30 mM NaCl (pH 7.4), and eluted at a flow rate of 0.4 ml min −1 . Fractions eluting between 9 and 11 ml were collected, and Reelin concentration was estimated by Bradford assay (Bio-Rad) using BSA as a protein standard. In parallel to Reelin, Mock supernatants were produced from 293T cells stably transfected with GFP [44] and subjected to the same purification protocol. Aβ 42 purification Aβ 42 was synthesized and purified by Dr James I. Elliott at Yale University (New Haven, CT, USA). The lowest aggregation state in which Aβ 42 can be prepared corresponds to LMW Aβ 42 , which contains monomer in rapid equilibrium with low- n Aβ oligomer forms, where n is the order of the oligomer. A LMW Aβ 42 preparation was obtained using size exclusion chromatography. Aβ peptide was dissolved in 6 M Gdn·HCl at 5 mg ml −1 , sonicated for 5 min, centrifuged at 10,000 g for 6 min, and passed through a 0.45-μm Millex filter. The resulting solution was injected into a Superdex 75 HR 10/300 column (GE Healthcare) previously equilibrated using 10 mM phosphate (pH 7.4), and eluted at a flow rate of 0.5 ml min −1 . The peak attributed to LMW Aβ 42 , eluted between 13 and 15 ml, was collected and its concentration was determined by Bradford assay. Aggregation studies Freshly purified Aβ 42 was diluted to 24 μM (108 ng μl −1 ) in 10 mM PB/5 mM NaCl (pH 7.4) and left to aggregate at 20 °C, alone or in the presence of purified Reelin. Freshly purified Reelin, quantified by Bradford assay, was diluted to reach a 6:1 w / w Aβ 42 :Reelin ratio (corresponding to 18 ng μl −1 of Reelin). As for Reelin, equivalent Mock volumes were left to aggregate with Aβ 42 . Reelin and Mock preparations without Aβ 42 were used as controls. Aggregation was monitored in parallel for the following aggregating solutions: Aβ 42 , Aβ 42 /Mock, Aβ 42 /Rln, Rln and Mock. Aliquots were taken from each solution every 24 h for the assays described below. ThT assays Aβ 42 , Aβ 42 /Mock, Aβ 42 /Rln, Rln and Mock aggregating solutions were subjected to ThT-binding assay by mixing 62.5 μl of each with 15 μl of ThT dye (100 μM) and 16.6 μl of 300 mM glycine NaOH at pH 8.5. The ThT-binding assay was performed in Hard Shell Thin Wall 96-well fluorescence plates (Bio-Rad). The ThT fluorescence of each sample was measured in a FluoDiaTM T70 fluorometer (Photon Technology International) at excitation and emission wavelengths of 450 and 485 nm, respectively. The samples were analysed in triplicate and average fluorescence values and s.d. were plotted. To determine the effect of Reelin on fibril formation, raw data obtained for the different aggregating solutions were fitted by a sigmoidal curve described by Eqn (1) using GraphPad Prism software, as described previously [38] , [45] : Y is the fluorescence intensity, t is time, t 0.5 is the time to 50% of maximal fluorescence, b is the slope, and top and bottom values correspond to the maximum and minimum fluorescence intensities. Estimated lag time is t 0.5 −2 b in each condition. Transmission electron microscopy A 10-μl aliquot of the samples subjected to aggregation studies was applied to a 200-mesh carbon-coated formvar grid, previously glow-discharged for 5 min. After 1 min, the grid was washed with water and negatively stained by treatment with 2% uranyl acetate for 1 min. Samples were observed in a JEOL JEM 1010 transmission electron microscope operating at 80 kV. Photo-induced crosslink of unmodified proteins PICUP reaction was based on detailed descriptions given in the literature [29] , [46] . The set-up consisted of a camera body and a 150-W slide projector. A PCR tube containing the reaction mixture to be crosslinked, subjected by a glass vial, was placed inside the camera body for irradiation. The sample was irradiated by means of the 150-W slide projector, precisely controlled by the camera shutter. PICUP reactions were carried out using an Aβ 42 :Ru(bpy) 3 2+ :APS ratio of 1:2:40. To this end, 0.8 μl of 1 mM Ru(bpy) 3 2+ and 0.8 μl of 20 mM APS were added to 18 μl of 24 μM Aβ 42 , Aβ 42 /Mock and Aβ 42 /Rln in 10 mM PB/30 mM NaCl (pH 7.4). The mixture was irradiated for 4 s at a distance of 25 cm and immediately quenched by adding 5 μl of 0.3 M DTT to the sample. Sample buffer (10 μl, 3 × ) was added to 20 μl of the sample to be analysed by SDS-PAGE. Samples were boiled at 95 °C for 5 min and analysed by western blot using 6E10 as primary antibody. Dot blot To analyse the oligomer content during the time-course of aggregation, 3 μl aliquots of Aβ 42 /Mock and Aβ 42 /Rln samples were applied to a nitrocellulose membrane. Membranes were processed as for western blot, using A11 as primary antibody. Immunogold labelling A 10-μl aliquot of the samples subjected to aggregation studies was applied for 3 min to a carbon-coated nickel formvar grid, previously glow-discharged for 5 min. Grids were then blocked three times for 5 min with FBS 10% in PB saline (PBS) 0.1 M. Primary antibodies were dissolved in a FBS 5% solution in PBS 0.1 M and applied for 30 min. The grids were then rinsed with 1% FBS in PBS 0.1 M and incubated with colloidal gold-coated secondary antibodies in a 5% FBS solution in PBS 0.1 M for 30 min. After washing, grids were fixed for 5 min with 2% glutaraldehyde and negatively stained with 2% uranyl acetate for 1 min. Samples were observed as for TEM. X-ray diffraction Aligned fibrils of Aβ 42 /Rln and Aβ 42 /Mock samples were prepared by suspending a 5-μl drop of aged fibril solution between two glass rods with beeswax tips ~1.5 mm apart. Before complete drying of the first drop, sequential addition of extra drops of 5 μl was performed twice. Finally, fibrils were allowed to dry completely. Fibril diffraction data were collected on a crystallography beamline at the University of Cambridge. Azimutal plots from diffractions were represented using ImageJ software. ADDLs preparation ADDLs were prepared as described [47] . Briefly, Aβ 42 was dissolved in hexafluoro-2-propanol (1 mg ml −1 ), aliquoted in low-binding Eppendorf tubes, and then hexafluoro-2-propanol was removed by freeze-drying. An aliquot of Aβ 42 was dissolved in anhydrous dimethyl sulfoxide (DMSO) to 5 mM and further diluted with ice-cold F12 medium without phenol red to 100 μm. This solution was incubated at 4 °C for 24 h and then centrifuged at 14 000 g for 10 min. The Aβ 42 concentration in the supernatant was determined using Bradford assay and found to range between 60 and 100 μM. The peptide solution was diluted to the desired concentrations for co-immunoprecipitation assays (10 μM) or for PI staining (3, 5 and 10 μM). Primary hippocampal cultures Hippocampal neurons were obtained from E16 OF1 mouse embryos (Charles River Laboratories). Brains were dissected in PBS containing 0.6% glucose, and hippocampi were excised. After trypsin (GIBCO) and DNAse (Roche Diagnostics) treatments, hippocampi were dissociated by gentle sweeping. Cells were counted and seeded onto poly- D -lysine-coated dishes in Neurobasal medium containing B27 supplement (GIBCO). Treatments were performed 72–96 h after cell seeding. Testing Reelin biological activity Primary hippocampal neurons seeded at 10 6 cells per well in six-well plates were treated with Reelin at a working concentration of 2–5 ng μl −1 (Mock samples were used in equivalent volumes). After 15 min, lysates were collected in lysis buffer (Hepes 50 mM (pH 7.5), 150 mM sodium chloride, 1.5 mM magnesium chloride, 1 mM EGTA, 10% glycerol and 1% Triton X-100) containing Complete Mini protease inhibitor cocktail (Roche) and phosphatase inhibitors (10 mM tetra-sodium pyrophosphate, 200 μM sodium orthovanadate and 10 mM sodium fluoride); insoluble debris was removed by centrifugation (30 min, 16,000 g ). To detect Dab1 phosphorylation, lysates were incubated with the primary antibody for immunoprecipitation overnight (o/n) at 4 °C. Protein G Sepharose beads were added for 90 min at 4 °C, recovered by centrifugation and washed three times with lysis buffer. Immunoprecipitated samples or their supernatants (used as loading controls) were diluted 1:6 with 6 × loading buffer (0.5 M Tris–HCl (pH 6.8), 2.15 M β-mercaptoethanol, 10% SDS, 30% glycerol and 0.012% bromophenol blue), boiled for 5 min at 95°C and processed for western blot. Reelin interaction with soluble Aβ 42 species Co-immunoprecipitation experiments for Aβ 42 and Reelin during the pre-fibrillar phase of the aggregation were performed in two independent experimental conditions: (1) using 40–80 μl of Aβ 42 /Rln sample from a very early stage of the in vitr o aggregation experiment (days 2–4) and (2) from 100 μl of ADDLs preparation (10 μM) mixed with Reelin (10 ng μl −1 ) in neurobasal medium and incubated for 1 h at 37 °C. In both conditions lysis buffer (Hepes 50 mM (pH 7.5), 150 mM sodium chloride, 1.5 mM magnesium chloride, 1 mM EGTA, 10% glycerol and 1% Triton X-100) was added to the samples up to 500 μl, and the mixtures were incubated with the required immunoprecipitation antibody for 1 h at 4 °C. Insoluble debris was removed by centrifugation (10 min, 16,000 g ) and supernatants incubated with Protein A and Protein G Sepharose 4 Fast Flowbeads for 90 min at 4 °C, recovered by centrifugation and washed three times with lysis buffer. Immunoprecipitated samples or their supernatants (used as loading controls) were diluted 1:6 with 6 × loading buffer, boiled for 5 min at 95 °C and processed for western blot. A diversity of control samples were processed in parallel including either Reelin or Aβ 42 (condition 1) or ADDLs (condition 2) alone. Negative controls without addition of antibody were also carried out in each experimental condition. Western blot Samples were resolved by SDS-polyacrylamide gels and transferred onto nitrocellulose membranes. Membranes were blocked for 1 h at room temperature (RT) in TBST (Tris 10 mM (pH 7.4), sodium chloride 140 mM (TBS) with 0.1% Tween 20) containing 5% non-fat milk or 3% BSA. Primary antibodies were incubated for 90 min in TBST–0.02% azide. After incubation with HRP-labelled secondary antibodies for 1 h at RT in TBST–5% non-fat milk, membranes were developed with the ECL system (GE Healthcare). PI staining Primary hippocampal neurons seeded at 10 5 cells per well in four-well plates containing coverslips were treated with ADDLs (3, 5 and 10 μM) or corresponding volumes of vehicle (0.1% DMSO in F12 medium), with or without the addition of Reelin at 5 ng μl −1 (or equivalent volumes of Mock). After 24 h, cells were incubated for 30 min with PI (1.5 μg ml −1 ) and Hoechst 33342 (1 μg ml −1 ) for counterstaining. Cells were washed three times with PBS and fixed for 20 min with 4% paraformaldehyde (PF) in 0.1 M PB. Fluorescent micrographs were randomly taken from coverslips for each condition. Number of dying neurons (PI and Hoechst double-labelled picnotic nuclei) versus total number of cells (Hoechst-labelled) per field were counted for statistics. Histological plaque staining Animals were anaesthetized and perfused for 20 min with PB-4% PF. Brains were removed, post-fixed overnight with PB–4% PF, cryoprotected with PB-30% sucrose and frozen. Brains were sectioned coronally (30 μm) and sections were blocked for 2 h at RT with PBS containing 10% of normal goat serum (NGS), 0.2% of gelatin and F(ab′)2 fragment anti-mouse IgG (1:300). Plaque-specific primary antibody (3D6) was incubated overnight at 4 °C with PBS-5% NGS. Sequential incubation with biotinylated secondary antibody (2 h at RT) and streptavidin-HRP (1:400; 2 h at RT) was performed in PBS–5% NGS. Bound antibodies were visualized by reaction using DAB and H 2 O 2 as peroxidase substrates. Sections were dehydrated and mounted (Eukitt). Golgi staining For Golgi–Colonnier staining, adult mice ( n =3 per group) were deeply anaesthetized and transcardially perfused with 2% PF–2% glutaraldehyde in 0.12 M PB. Brains were removed from the skull and post-fixed in the same solution overnight. Pieces containing the whole hippocampal formation were excised and incubated in a dichromate–Colonnier solution (3% K2Cr2O7, 5% glutaraldehyde in H2O) for 5 days at 15 °C. Pieces were transferred to a 0.75% AgNO3 solution for 3 days. After embedding in paraffin, 200-μm thick sections were obtained and subsequently dehydrated. The sections were then mounted onto slides and coverslipped with an Araldite solution. Novel object recognition The NOR task was performed in groups of 8–12 males per genotype (control; TgRln; J20; TgRln/J20). Mice were individually placed in an L-shaped maze (equal arms of 15 × 5 cm) with grey, non-reflective base plate for 15 min (day 0, habituation phase). The next day, animals were exposed to two identical elements (located at the edge of each arm) for 15 min (day 1, acquisition phase). The following day, mice were returned to the maze that now contained one known and one novel object (day 2, recognition phase). The type and positions of the known and novel objects in the chamber were changed semi-randomly between mice but kept constant for any given animal. The time that mice spent exploring each of the two objects in the acquisition and recognition phases was measured. The discrimination index for the novel object was calculated as the time exploring the novel object minus the time exploring the known object, relative to total time exploring (exploration of old and new object). Statistical analysis To determine plaque load in the hippocampus (from 1.35–2.30 mm posterior to Bregma) and in the entorhinal cortex the area immunostained with plaque-specific antibody was determined using ImageJ software and normalized to the total hippocampal area. Significance between groups (J20; TgRln/J20) was analysed for each area using the unpaired Student’s t -test ( n =3–5 animals per group; 6–8 sections per animal). To quantify toxicity from the PI-stained cell cultures, fluorescent micrographs were randomly taken from coverslips for each condition. The number of dying neurons versus total number of cells per field were counted for statistics from four independent experiments ( n =15–40 fields per condition). Percentage of survival (%survival) per field was calculated following Equation (2): %field is the percentage of dead cells in a specific field; vehicle is the average percentage of dead cells per field in vehicle-treatment conditions in a specific experiment; triton is the average percentage of dead cells in 0.01% triton X-100-treatment conditions in a specific experiment. Significance was analysed by one-way ANOVA. Orthogonal comparisons of Mock versus Reelin treatments for each concentration of ADDLs were analysed with the unpaired Student’s t -test. Spine density from Golgi-stained preparation was counted at hippocampal area over 10 μm in secondary dendrites from the stratum radiatum and the stratum lacunosum moleculare of CA1 pyramidal neurons starting at 5–10 μm from the ramification point ( n =3 animals per group; 20–35 neurons). Significance was analysed by one-way ANOVA. Orthogonal comparisons of J20 versus TgRln/J20 for each brain area were analysed with the unpaired Student’s t -test. To determine differences in NOR task between groups, discrimination indexes were analysed. Significance was analysed by one-way ANOVA. Orthogonal comparisons of J20 versus TgRln/J20 and control versus TgRln for each age were analysed with the unpaired Student’s t -test. How to cite this article: Pujadas, L. et al . Reelin delays amyloid-beta fibril formation and rescues cognitive deficits in a model of Alzheimer’s disease. Nat. Commun. 5:3443 doi: 10.1038/ncomms4443 (2014).